Attosecond tracing of correlated electron-emission in non-sequential double ionization Despite their broad implications for phenomena such as molecular bonding or chemical reactions, our knowledge of multi-electron dynamics is limited and their theoretical modelling remains a most difficult task. From the experimental side, it is highly desirable to study the dynamical evolution and interaction of the electrons over the relevant timescales, which extend into the attosecond regime. Here we use near-single-cycle laser pulses with well-defined electric field evolution to confine the double ionization of argon atoms to a single laser cycle. The measured two-electron momentum spectra, which substantially differ from spectra recorded in all previous experiments using longer pulses, allow us to trace the correlated emission of the two electrons on sub-femtosecond timescales. The experimental results, which are discussed in terms of a semiclassical model, provide strong constraints for the development of theories and lead us to revise common assumptions about the mechanism that governs double ionization. Many fundamental processes in nature such as the formation and dissociation of molecules are governed by multi-electron dynamics (MED). Understanding MED is one of the grand contemporary challenges of quantum physics. While the ground state properties of multi-electron systems are described with reasonable accuracy, the modelling of their dynamics is still in its infancy. Even for rather simple systems involving only a few interacting electrons such as low-Z atoms beyond helium (Z being the nuclear charge), the exact theoretical treatment of MED is hardly practicable. The identification of suitable approximations that capture the essential features of MED relies on the development of experiments aimed at resolving the electron dynamics on the characteristic attosecond timescale of their motion. An established technique for resolving one-electron dynamics on sub-femtosecond scales involves the use of a strong few-cycle infrared laser field as a clock [1] , [2] , [3] . The well-known concept of attosecond streaking spectroscopy has permitted the observation of single-electron dynamics with attosecond time resolution [4] . Despite this progress, however, the ultrafast dynamics of multiple electrons has resisted direct observation, even though far-reaching conclusions were drawn from kinematically complete strong-field double [5] , [6] and multiple ionization [7] experiments. Among countless phenomena involving the motion of multiple electrons, non-sequential double ionization (NSDI) of atoms is a pure and, meanwhile, classic example for MED in the presence of strong fields. As reported for rare gases almost 30 years ago [8] , it manifests itself as an unexpected, orders-of-magnitude enhancement in the strong-field double ionization yield. This finding cannot be explained within the framework of the single active electron approximation, where both electrons are assumed to be ionized sequentially and independently of each other. A mechanism correlating the emission of the two electrons must be included to adequately describe this effect and different models have been proposed [5] , [9] . Since the pioneering works, NSDI has been the subject of numerous experimental and theoretical studies (for a recent review, see ref. 6 and references therein). Recording the momentum spectra of doubly [10] , [11] and multiply [7] charged ions provided clear evidence that the emission of the second electron is triggered by the laser-driven recollision of the first electron with its parent ion. Even more insight into the process was gained in kinematically complete studies where the correlated two-electron momentum distributions were measured [11] and investigated for different laser parameters [12] , [13] , [14] , [15] . Measurements of the dynamics of NSDI in near-single cycle laser pulses have been restricted to recoil-ion spectra, which did not allow for the direct retrieval of the correlated electron-emission dynamics [16] , [17] . The sub-cycle dependence of electron correlation spectra has been explored by various theoretical studies, where the double-ionization dynamics were confined to a single cycle of a laser pulse [12] , [18] . A direct test of the validity of these theoretical models, however, has been impeded so far by the lack of kinematically complete experimental data obtained with ultrashort pulses and precise control or knowledge of the electric field. Here we present measurements of correlated two-electron momentum spectra for the strong-field NSDI of argon atoms in the single-cycle limit. The measured spectrum exhibits a cross-shaped structure that qualitatively differs from spectra recorded in all previous experiments using many-cycle pulses. Confining the ionization dynamics to a single laser cycle by choosing an adequate carrier envelope phase (CEP) allows us to perform a clean experiment with only one single recollision event contributing to NSDI, thus excluding the contribution of multiple recollisions that hamper the interpretation of experimental results. From the CEP-resolved spectra the correlated emission of two electrons is traced on sub-femtosecond timescales. In particular, we can determine at which time the second electron is released within the laser pulse. Experimental set-up A detailed sketch of our experimental set-up is given in the Methods. Briefly, the experiments were performed using linearly polarized laser pulses with a central wavelength of 750 nm and a full-width at half-maximum (FWHM) of the temporal intensity envelope of 4 fs, which were generated at a repetition rate of 3 kHz [19] . The electric field of the laser pulse can be approximated as E ( t )= E 0 cos 2 ( t/τ ) cos(ω t + φ ), where E 0 is the field amplitude, ω is the carrier frequency, τ is the pulse duration, and φ is the CEP. Combining a reaction microscope (REMI) [20] with a newly developed phase-tagging technique [21] , we obtained the CEP of the laser pulse for each and every ionization event [22] recorded with the REMI. The laser was focussed to a maximum instantaneous intensity of into a cold supersonic gas jet of neutral argon atoms located in the centre of the REMI. The momenta of electrons and ions created in the laser focus were measured in coincidence in the REMI. For the conditions of our experiment, the ratio of the measured Ar 2+ to Ar + yields was about 0.1%. 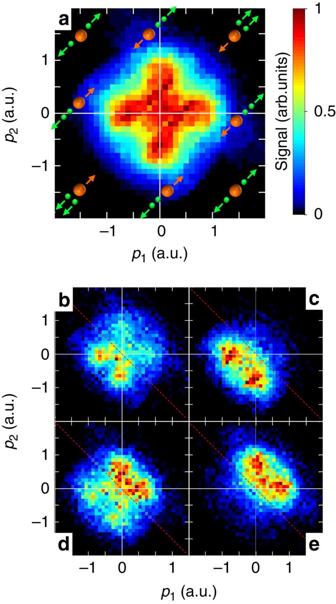Figure 1: Correlated two-electron momentum spectra. Experimental two-electron momentum distributions for the double ionization of argon with near-single cycle, 4 fs laser pulses at a maximum instantaneous intensity ofI0=3.0×1014Wcm−2. Herep1andp2are the momentum components of the first and the second electron along the laser polarization direction, respectively. The cartoons in (a) illustrate the emission direction of the two electrons (green spheres) and the ion (orange spheres). The arrows represent the sign of the longitudinal momentum of the fragments. An event in the first or third quadrant corresponds to the emission of two electrons into the same direction; electrons emitted in opposing directions appear in the second or fourth quadrant. A cross-shaped structure is seen in the phase-integrated plot (a), reflecting the correlated nature of the NSDI process. In images (b–e), spectra are shown for different values of the CEP, namely (b) 65°, (c) 155°, (d) 245° and (e) 335°. The spectra are averaged over aπ/6 CEP range and are symmetrized with respect to thep2=p1diagonal. Images (c,e) correspond to CEPs with maximum asymmetry in the Ar2+emission and (b,d) to CEP with zero asymmetry in the Ar2+emission. The same colour scale is used for all (a–e). Two-electron momentum distributions Figure 1 shows experimental correlated two-electron momentum distributions, where the number of recorded double-ionization events is plotted as a function of the momenta p 1 and p 2 along the laser polarization axis of electron 1 and electron 2, respectively. The spectra are symmetric with respect to the p 2 = p 1 diagonal because the two electrons, the recolliding electron and the one liberated as a result of this recollision, cannot be distinguished in the experiment. The CEP-averaged correlation spectrum is shown in Fig. 1a . The cross-shaped structure indicates that the momentum of one electron is always close to zero whereas the momentum of the other electron varies between −1.5 to 1.5 atomic units. Similar structures were found in a recent theoretical study on NSDI of argon employing S-matrix theory [18] . So far, however, such a cross-shaped two-electron momentum distribution has not been observed experimentally. This strongly suggests that the physical mechanisms that govern NSDI in the near single-cycle regime differ from the many-cycle regime, where previous experiments were performed. The CEP-resolved correlation spectra presented in Fig. 1b–e exhibit a strong CEP dependence. For CEP values of 155° ( Fig. 1c ) and 335° ( Fig. 1e ), the signal is predominantly (with more than 80% of the counts) located below and above the red diagonal line ( p 2 =− p 1 ), respectively. For intermediate CEP values of 65° ( Fig. 1b ) and 245° ( Fig. 1d ), the signal is distributed on both sides of the red diagonal. Figure 1: Correlated two-electron momentum spectra. Experimental two-electron momentum distributions for the double ionization of argon with near-single cycle, 4 fs laser pulses at a maximum instantaneous intensity of I 0 =3.0×10 14 Wcm −2 . Here p 1 and p 2 are the momentum components of the first and the second electron along the laser polarization direction, respectively. The cartoons in ( a ) illustrate the emission direction of the two electrons (green spheres) and the ion (orange spheres). The arrows represent the sign of the longitudinal momentum of the fragments. An event in the first or third quadrant corresponds to the emission of two electrons into the same direction; electrons emitted in opposing directions appear in the second or fourth quadrant. A cross-shaped structure is seen in the phase-integrated plot ( a ), reflecting the correlated nature of the NSDI process. In images ( b–e ), spectra are shown for different values of the CEP, namely ( b ) 65°, ( c ) 155°, ( d ) 245° and ( e ) 335°. The spectra are averaged over a π /6 CEP range and are symmetrized with respect to the p 2 = p 1 diagonal. Images ( c , e ) correspond to CEPs with maximum asymmetry in the Ar 2+ emission and ( b , d ) to CEP with zero asymmetry in the Ar 2+ emission. The same colour scale is used for all ( a – e ). Full size image The semiclassical model To interpret the experimental results, we investigate the recollision-induced ionization dynamics using a semiclassical model (for details, see Methods). In the present intensity regime, essentially two mechanisms may contribute: the first is the (e, 2e)-mechanism, in which the recolliding electron directly promotes a second electron into the continuum via electron impact ionization [23] . The second is recollision-induced excitation with subsequent ionization (RESI) [24] , [25] , where the recolliding electron excites the parent ion, which is subsequently ionized by the laser field as depicted in Fig. 2a . A key property of the RESI process is the delayed emission of the second electron with respect to the recollision event, the latter occurring near the zero crossing of the electric field of the laser. As shown below, our experimental results identify RESI as the dominant process, and, more importantly, enable the determination of the emission delay. 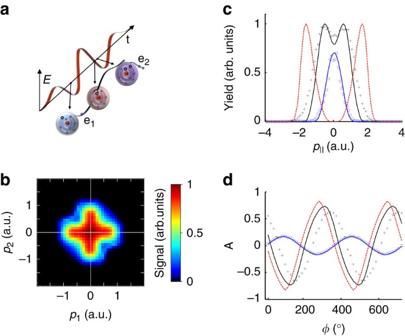Figure 2: Comparison of experimental and theoretical results. (a) Illustration of the RESI mechanism dominating NSDI at the experimental parameters: the laser electric field as a function of time is drawn along with schematics of the electronic configuration of the outer shell of Ar at three key time steps of the process. First, an electron e1is liberated from Ar, leaving a hole (small circle) in the outer shell of Ar+(light blue). Second, an excited Ar+ion (pink colour) is produced upon recollision of electron e1near the zero-crossing of the electric field. Finally, a second electron e2is liberated from the excited Ar+ion forming Ar2+(purple). (b) Calculated two-electron momentum spectrum averaged over CEP for the experimental parameters using the semiclassical RESI model, described in the text. (c) Experimental recoil-ion momentum spectra (for momentap||parallel to the polarization axis) for single (Ar+ions, blue open dots) and double ionization (Ar2+ions, black crosses), respectively, averaged over CEP. The experimental data are compared with the model results for single ionization (blue line), and double ionization ((e, 2e)-mechanism (dashed red line) and RESI-mechanism (black line)). Scattering anglesβ=0° andβ=20° are used to simulate the (e, 2e) and RESI processes, respectively. (d) Comparison of the experimental and calculated asymmetryAas a function of the CEPφfor Ar+and Ar2+(using the same symbols and colour coding as in (c)). All the theoretical results shown in (b,c,d) were obtained from the same simulation with the parameters given in the text. Figure 2: Comparison of experimental and theoretical results. ( a ) Illustration of the RESI mechanism dominating NSDI at the experimental parameters: the laser electric field as a function of time is drawn along with schematics of the electronic configuration of the outer shell of Ar at three key time steps of the process. First, an electron e 1 is liberated from Ar, leaving a hole (small circle) in the outer shell of Ar + (light blue). Second, an excited Ar + ion (pink colour) is produced upon recollision of electron e 1 near the zero-crossing of the electric field. Finally, a second electron e 2 is liberated from the excited Ar + ion forming Ar 2+ (purple). ( b ) Calculated two-electron momentum spectrum averaged over CEP for the experimental parameters using the semiclassical RESI model, described in the text. ( c ) Experimental recoil-ion momentum spectra (for momenta p || parallel to the polarization axis) for single (Ar + ions, blue open dots) and double ionization (Ar 2+ ions, black crosses), respectively, averaged over CEP. The experimental data are compared with the model results for single ionization (blue line), and double ionization ((e, 2e)-mechanism (dashed red line) and RESI-mechanism (black line)). Scattering angles β =0° and β =20° are used to simulate the (e, 2e) and RESI processes, respectively. ( d ) Comparison of the experimental and calculated asymmetry A as a function of the CEP φ for Ar + and Ar 2+ (using the same symbols and colour coding as in ( c )). All the theoretical results shown in ( b , c , d ) were obtained from the same simulation with the parameters given in the text. Full size image In our semiclassical model, the probability to liberate the first electron at any moment in time is calculated using the instantaneous Ammosov–Delone–Krainov (ADK) tunnelling rate including a correction factor to account for over-the-barrier ionization [26] . The propagation of the electron after the ionization in the electric field of the laser pulse is treated classically, neglecting the Coulomb interaction with the ionic core and with the other electron. For the RESI process, the calculation is performed as follows: if the first electron recollides with the parent ion with sufficient kinetic energy, the lowest excited state of Ar + is populated and the second electron is liberated by subsequent field ionization. For the (e, 2e) process, we consider only recolliding electrons having sufficient energy to overcome the second ionization potential of argon. In this case, the second electron is assumed to be liberated with zero-initial momentum via electron impact ionization. In both the RESI and (e, 2e) processes, the magnitude of the first electron momentum, just after the recollision, is determined by energy conservation. The direction of this momentum vector, described by the scattering angle β (where β is the angle between the momentum vectors just before and just after the recollision), is undetermined in our model and constitutes the only free parameter. The dependence of the simulated correlation spectra on the scattering angle is discussed in the Methods. Comparison of measured and calculated spectra The results of our calculations are displayed in Fig. 2b–d , for the instantaneous peak intensity of I 0 =2.9×10 14 Wcm −2 (the cycle-averaged peak intensity equals I 0 /2) and a pulse duration of 3.8 fs (FWHM in intensity). In Fig. 2c , the measured CEP-averaged momentum distributions of Ar + and Ar 2+ are compared with their simulated counterparts for the (e, 2e) and RESI mechanisms. The calculated width of the Ar + spectrum is in good agreement with the measurement. The double hump structure of the Ar 2+ spectrum is also correctly reproduced by the simulation for the RESI mechanism, where the best agreement was reached with β =20°. We note that small contributions of higher excited Ar + states or the (e, 2e) mechanism would lead to a slightly broader momentum distribution of the Ar 2+ ions in the calculations. The prediction for the (e, 2e) mechanism alone (red line in Fig. 2c ), however, does not reproduce the experimental Ar 2+ spectrum even if we use β =0°, where the best agreement was reached for this mechanism. Interestingly, the double hump structure, which was previously believed to originate from an (e, 2e) mechanism [27] can be reproduced considering the RESI mechanism only. Figure 2b shows the calculated CEP-averaged correlation spectrum for the RESI process, which exhibits the characteristic cross-shaped structure observed in the experiment. The corresponding two-electron momentum distribution for the (e, 2e) process is shown for comparison in the Methods. Comparison of measured and calculated asymmetries In earlier work, the (e, 2e) mechanism was invoked to explain the CEP-dependent Ar 2+ recoil-ion spectra at about twice the intensity [16] , [28] . Our results clearly indicate that, under the conditions of the present experiment, electron impact excitation to the lowest excited Ar + state and subsequent field ionization (RESI) constitutes the main contribution to NSDI of argon. To discuss the CEP dependence of NSDI, it is instructive to introduce the asymmetry parameter A =( N + − N − )/( N + + N − ), where N + and N − denote the number of ions with positive and negative momentum along the polarization axis, respectively. In Fig. 2d , the measured asymmetries of the Ar + and Ar 2+ yields as a function of CEP are compared with the results of our calculations (using the parameters given above). The experimental CEP is only determined up to a constant offset (see Methods). We use the theoretical Ar + asymmetry as a reference to set the value of the offset such that the maximum of the measured Ar + asymmetry curve coincides with the maximum of the calculated one. Remarkably, both the amplitude and the shape of the simulated Ar + asymmetry curve exactly match the measurement. Whereas the amplitudes of the calculated and measured Ar 2+ asymmetry curves are in good agreement, the calculated phase shifts between the Ar + and the Ar 2+ asymmetry curves (154° for RESI and 177° for (e, 2e)) do not match the measured phase shift of 114°. We would like to emphasize that such asymmetry data obtained simultaneously for single and double ionization is only accessible in the few and near single-cycle regime and was not available before. The measured phase shift represents a useful observable to test the validity of theoretical models. In spite of the small discrepancies between the experimental data and the simulation results, the overall agreement is impressive, considering the simplicity of the theoretical model. In light of the good agreement between simulation and experiment, the electron dynamics can now be analysed in more detail. In Fig. 3 , experimental ( Fig. 3a,b ) and simulated ( Fig. 3c,d ) correlation spectra are compared for CEP values that correspond to maximum ( Fig. 3a,c ) and zero ( Fig. 3b,d ) Ar 2+ asymmetry, respectively. Figures 3e and 3f show the calculated ionization rates of the first (green area) and second (red area) electron together with the temporal profile of the laser electric field for these two CEP values. Due to depletion of the excited Ar + population, the second electron is emitted before the maximum of the laser electric field. Our analysis thus reveals that under our experimental conditions, it is the momentum of the first electron that is close to zero while the momentum of the second electron is non-zero and varies as a function of the CEP. Averaged over the CEP, this results in the cross-shaped structures seen in Figs 1a and 2b . This finding is in contrast to the common assumption that the second electron in the RESI mechanism is released at the peak of the electric field and acquires a small momentum distributed around zero [7] . 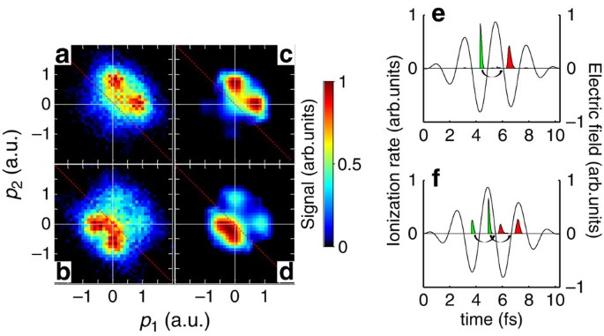Figure 3: Timing of the first and second ionization. Comparison of measured (a,b) and calculated (c,d) two-electron momentum distributions for CEPs corresponding to a maximum (a,c) and zero value (b,d) of the Ar2+asymmetry. The predicted ionization rates of the first (green-shaded area) and second (red-shaded area) electron contributing to NSDI are displayed in (e) and (f) together with the electric field of the laser pulse (black line) for maximum and zero Ar2+asymmetry parameters, respectively. Each black arrow points to the time of recollision for electrons liberated near the tail of the arrow. In (a,c,e) only a single recollision leads to NSDI, while in (b,d,f) two recollision events in successive half-cycles contribute. Figure 3: Timing of the first and second ionization. Comparison of measured ( a,b ) and calculated ( c,d ) two-electron momentum distributions for CEPs corresponding to a maximum ( a , c ) and zero value ( b , d ) of the Ar 2+ asymmetry. The predicted ionization rates of the first (green-shaded area) and second (red-shaded area) electron contributing to NSDI are displayed in ( e ) and ( f ) together with the electric field of the laser pulse (black line) for maximum and zero Ar 2+ asymmetry parameters, respectively. Each black arrow points to the time of recollision for electrons liberated near the tail of the arrow. In ( a , c , e ) only a single recollision leads to NSDI, while in ( b , d , f ) two recollision events in successive half-cycles contribute. Full size image Multiple recollision events, which occur in the several-to-multi-cycle regime, severely hamper the interpretation of measured correlation spectra. Figure 3 illustrates how the short pulses used in our study allow for a clean experiment by confining NSDI to essentially one single recollision event for an appropriate choice of the CEP yielding the maximum Ar 2+ asymmetry. For a CEP corresponding to a zero Ar 2+ asymmetry ( Figs 3b and d ), precisely two recollision events from consecutive half-cycles contribute to NSDI. Here the second electron, liberated as a result of the first recollision, acquires a higher momentum with positive sign whereas the second recollision results in a lower momentum with negative sign. Even in this case, the change in sign of the slope of the electric field allows for distinguishing the contributions from the two consecutive recollision events. With the analysis presented in Fig. 3, we can also unambiguously determine whether excitation of the singly charged ion occurs without recollision, that is, via laser excitation alone. Recollision-induced excitation takes place about three quarters of a cycle after the emission of the first electron. In contrast, a laser-excited ion would be efficiently ionized in the half-cycle following ionization of the first electron, leading to a signal on either side of the red diagonal in Fig. 3a , which is not observed. Disentangling laser excitation from recollisional excitation is possible only because the double ionization process has been confined to a single cycle. Using the infrared field as an inherent clock and neglecting the effect of the Coulomb potential as commonly assumed in the attosecond streaking scenario [1] , [29] , we can retrieve the electron's most likely emission time, which is directly mapped onto its drift momentum. Specifically, Δ t =arccos( p 0 / p max )/ ω , where p 0 and p max are the most probable and the maximum momentum of electron 2, respectively. From the experimental data, we find the maximum emission probability of the second electron at 210±40 attoseconds before the peak of the half-cycle following the recollisional excitation. This is in good agreement with our simulations predicting the emission leading the maximum of the field by 230 attoseconds. In conclusion, using a near-single-cycle laser pulse with appropriate CEP, the double ionization dynamics of argon could be confined to an isolated recollision event, allowing us to investigate the elementary process responsible for NSDI. The measured correlated two-electron momentum spectrum has a cross-shaped structure, which has not been observed in previous experiments, all of them using longer laser pulses. This suggests that the transition from the multi-cycle to the near-single-cycle regime substantially modifies the dynamics of NSDI. Resolving the CEP-dependence of the correlated two-electron spectra has provided new insights into the double ionization dynamics. In particular, we have shown that, owing to depletion of the excited Ar + ions, the second electron is emitted before the maximum of the laser electric field. The mean delay between the zero crossing of the electric field and the emission of the second electron could be determined unambiguously. More generally, the highly differential data obtained in our experiment provide strong constraints to multi-electron theories and may greatly stimulate their development. Whereas our semiclassical model captures the essential features of the data, electron correlations enter the model only indirectly via the ionic excitation and the scattering angle. More sophisticated models accounting for Coulomb and exchange interaction are certainly needed to fully resolve the correlated electron motion and predict the correct value for the phase shift observed between the Ar + and Ar 2+ asymmetry curves. Extension of our approach to the study of molecular dynamics may give a more detailed insight into the breaking of chemical bonds. Experimental technique The experiment was performed at the AS-1 attosecond beamline at the Max Planck Institute of Quantum Optics [19] . Linearly polarized laser pulses with a central wavelength of 750 nm, an energy of 400 μJ and a FWHM of the temporal intensity envelope of 4 fs are generated at a repetition rate of 3 kHz in an amplified laser system. Active stabilization of the CEP is difficult to conciliate with the long data-acquisition times (32 h for the present experiment) imposed by coincident particle-detection schemes. As a significant advance over previous efforts to measure the sub-femtosecond dynamics of the NSDI of argon, we recorded the CEP of each laser pulse by sending a fraction of the laser beam (25 μJ) into a single-shot stereographic above-threshold ionization (Stereo-ATI) phase-meter [21] (see Fig. 4 ). 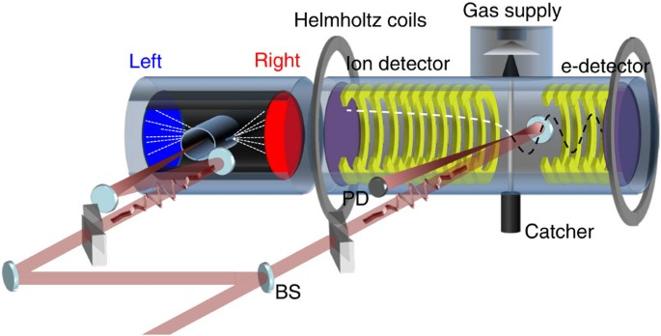Figure 4: Experimental set-up. Schematic of the set-up consisting of a single-shot Stereo-ATI phase meter (left chamber) and a REMI spectrometer (right chamber). A beamsplitter (BS) directs the laser pulses into both chambers. Each arm is equipped with a pair of fused-silica wedges for compensating residual chirp. The phase meter contains a layer of μ-metal to shield from external magnetic fields. The inner gas cell is filled with xenon gas at a pressure of about 5×10−3mbar. In the Stereo-ATI, xenon atoms are ionized near the focus of the horizontally polarized laser beam, and the electrons produced enter the high-vacuum drift tubes through slits. Electrons resulting from the ionization by a single-laser shot are detected by MCP detectors to the left and to the right, enabling the determination of the CEP for each REMI event, as described in the text. Simultaneously, ions and electrons created in the overlap of the laser focus and a skimmed supersonic jet of the REMI are extracted from the interaction region by a weak electric field (3 V cm−1) and detected by MCP and delay line detectors on the left and right side of the instrument, respectively. Helmholtz coils are used to facilitate the detection of electrons over a solid angle of 4π. The jet is efficiently pumped by the catcher. The master trigger for the electronics is provided by a fast photodiode (PD). The ion and electron optics are symmetric in reality, and a few electrodes have been removed for visualization of the laser path. Figure 4: Experimental set-up. Schematic of the set-up consisting of a single-shot Stereo-ATI phase meter (left chamber) and a REMI spectrometer (right chamber). A beamsplitter (BS) directs the laser pulses into both chambers. Each arm is equipped with a pair of fused-silica wedges for compensating residual chirp. The phase meter contains a layer of μ-metal to shield from external magnetic fields. The inner gas cell is filled with xenon gas at a pressure of about 5×10 −3 mbar. In the Stereo-ATI, xenon atoms are ionized near the focus of the horizontally polarized laser beam, and the electrons produced enter the high-vacuum drift tubes through slits. Electrons resulting from the ionization by a single-laser shot are detected by MCP detectors to the left and to the right, enabling the determination of the CEP for each REMI event, as described in the text. Simultaneously, ions and electrons created in the overlap of the laser focus and a skimmed supersonic jet of the REMI are extracted from the interaction region by a weak electric field (3 V cm −1 ) and detected by MCP and delay line detectors on the left and right side of the instrument, respectively. Helmholtz coils are used to facilitate the detection of electrons over a solid angle of 4 π . The jet is efficiently pumped by the catcher. The master trigger for the electronics is provided by a fast photodiode (PD). The ion and electron optics are symmetric in reality, and a few electrodes have been removed for visualization of the laser path. Full size image A detailed description of the CEP measurement technique using ATI and the Stereo-ATI phase meter can be found in refs 17 , 21 , 22 , 30 , 31 . Briefly, the time-of-flight spectra of electrons emitted along both directions of the laser polarization axis are recorded on either side of the apparatus (left and right detector in Fig. 4 ). For each laser shot, the CEP is inferred from the asymmetry between the left and the right TOF spectra. The CEP is measured up to a constant offset in the phase meter. A fraction (11 μJ) of the remaining part of the laser beam is focussed with a spherical mirror ( f =25 cm) into a well-localized (1 mm width) and cold supersonic gas jet of neutral argon atoms in the centre of a REMI [20] . Ions and electrons created in the laser focus (~40 μm diameter) are extracted by a weak electric field towards microchannel plate (MCP) detectors equipped with delay line anodes for position readout at the left and right side of the instrument, respectively. A pair of Helmholtz coils generates a homogenous magnetic field to guide the electrons towards their detector reaching a 4 π acceptance angle for all electrons of interest ( Fig. 4 ). The 3D momentum vectors of ions and electrons are reconstructed from their measured flight times and impact positions on the corresponding detectors. The low density of the jet allows for detection of on average less than one ionization event per laser shot, an important constraint to minimize the number of false coincidences, when measuring ions and electrons in coincidence. In the present experiment, 0.25 ions per laser shot were detected on average. Data processing and false coincidences To generate the correlated two-electron momentum distributions shown in Fig. 1, we select laser shots where at least one electron and one Ar 2+ ion are detected. As most of the time only one of the two electrons generated together with Ar 2+ is detected (because of the single-particle detection efficiency of ~50%), the momentum of the missing second electron is calculated using momentum conservation. Electrons emerging from single ionization of argon introduce a false coincidence background in the electron correlation spectra of less than 15%. The contribution of false Ar 2+ events (<0.5% of the total Ar 2+ signal) is negligible. Laser intensity and CEP offset measurement The analysis of the Ar + spectra, recorded in the same measurement, provides important information allowing for in situ determination of the peak intensity of the laser pulse in the interaction region, as shown in Fig. 5 . Furthermore, the comparison of the measured and calculated Ar + asymmetry curves allows for the determination of the absolute CEP of the laser pulses in the interaction region in the REMI. 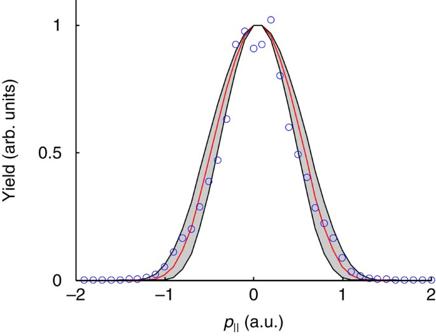Figure 5: Determination of the peak intensity. The peak intensity in the laser focus is inferred from the momentum spectra of Ar+ions (parallel to the polarization axis) by comparison with simulations. The measured Ar+spectrum (open circles) is plotted together with simulated spectra calculated for three different intensities: 3.0×1014W cm−2(red line), 2.4×1014W cm−2and 3.6×1014W cm−1(narrow and wide black spectra respectively). The gray area in-between the two black curves represents the error bars of ±20% in the determination of the peak intensity. Figure 5: Determination of the peak intensity. The peak intensity in the laser focus is inferred from the momentum spectra of Ar + ions (parallel to the polarization axis) by comparison with simulations. The measured Ar + spectrum (open circles) is plotted together with simulated spectra calculated for three different intensities: 3.0×10 14 W cm −2 (red line), 2.4×10 14 W cm −2 and 3.6×10 14 W cm −1 (narrow and wide black spectra respectively). The gray area in-between the two black curves represents the error bars of ±20% in the determination of the peak intensity. Full size image Simulation procedure The yield Y ( t ) of electrons emitted in a time interval [ t , t +d t ] is calculated using the instantaneous ADK tunnelling rate w ADK (refs 32 , 33 ) summed over all occupied degenerate states of the outer shell. This rate is further multiplied with the correction factor from (ref. 26 ) to account for above the barrier ionization: Here I p is the ionization potential and α is a numerical factor adjusted such that the rate, w ( t ), fits the result obtained by solving the Schrödinger equation numerically. The value of parameter α is 9 for Ar and 8 for Ar + (ref. 26 ). The ionization yield is calculated as where N ( t i ) is the initial population of the electronic state under consideration. After ionization, at time t 0 , the electron enters the continuum with zero momentum at a distance x t of the parent ion, where x t is the exit of the tunnel. The electron is propagated classically in the electric field of the laser pulse, neglecting the interaction with the parent ion. The electron may return at a later time t 1 , to the position at x 0 , with sufficient energy to either excite the parent ion in the case of RESI or to directly ionize the parent ion in the case of the (e, 2e)-mechanism. For the RESI process, the calculation is performed as follows: if the kinetic energy, E kin ( t 1 ) of the returning electron is higher than the excitation energy, E exc =13.5 eV, needed to reach the lowest excited state of Ar + , this state, (3 s 3 p 6 ) 2 S 1/2 , is populated with the probability Y( t 0 ) and the propagation of the re-scattered electron is continued with an initial kinetic energy E ′ kin ( t 1 )= E kin ( t 1 )− E exc . For the ionization of the second electron from the excited ion, we proceed in the same way as for the ionization of the first electron, using the parameters of the excited state for the ionization rate. To simulate the (e, 2e) process, a recolliding electron with sufficient energy to overcome the second ionization potential of argon is assumed to produce a second electron with zero-initial momentum. The magnitude of the first electron momentum just after the recollision is determined by energy conservation. As indicated in the main text, the experimental data cannot be described by our model assuming the (e, 2e) process. In addition to the predicted recoil-ion momentum spectrum and asymmetry curve presented in Fig. 2 , the two-electron correlation spectrum calculated assuming the (e, 2e) mechanism is shown in Fig. 6 . 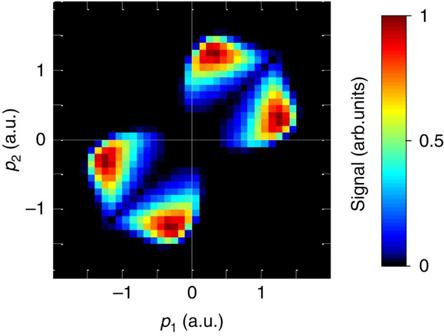Figure 6: Simulation results for electron impact ionization. Predicted two-electron momentum distribution for the (e, 2e) mechanism andβ=0°. The discrepancies between the (e, 2e) calculations and the measured data become even larger for other values ofβ. Figure 6: Simulation results for electron impact ionization. Predicted two-electron momentum distribution for the (e, 2e) mechanism and β =0°. The discrepancies between the (e, 2e) calculations and the measured data become even larger for other values of β . Full size image For both the (e, 2e) and RESI processes, the final drift momentum of the first electron depends on the scattering angle β (the angle between the momentum vectors just before and just after the recollision). The sensitivity of the simulation on the scattering angle is shown in Fig. 7 for the RESI process. We find that the cross-shaped structure is significantly altered if β is varied by±10 degrees. Focal volume averaging is taken into account by assuming a Gaussian intensity profile, neglecting the intensity variation across the argon gas jet of 1 mm diameter. 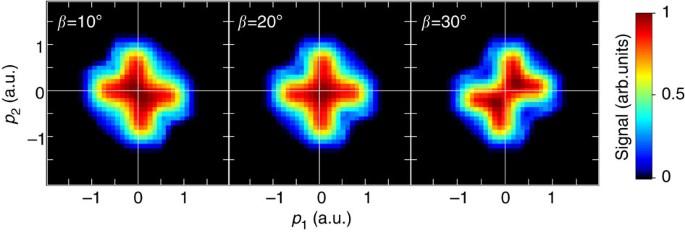Figure 7: Sensitivity with respect to the scattering angle. Simulated two-electron momentum distribution assuming the RESI process for three different scattering anglesβ. Figure 7: Sensitivity with respect to the scattering angle. Simulated two-electron momentum distribution assuming the RESI process for three different scattering angles β . Full size image How to cite this article: Bergues, B. et al . Attosecond tracing of correlated electron-emission in non-sequential double ionization. Nat. Commun. 3:813 doi: 10.1038/ncomms1807 (2012).